Asymmetric α-C(sp3)−H allylic alkylation of primary alkylamines by synergistic Ir/ketone catalysis Primary alkyl amines are highly reactive in N-nucleophilic reactions with electrophiles. However, their α-C−H bonds are unreactive towards electrophiles due to their extremely low acidity (p K a ~57). Nonetheless, 1,8-diazafluoren-9-one (DFO) can activate primary alkyl amines by increasing the acidity of the α-amino C−H bonds by up to 10 44 times. This makes the α-amino C−H bonds acidic enough to be deprotonated under mild conditions. By combining DFO with an iridium catalyst, direct asymmetric α-C−H alkylation of NH 2 -unprotected primary alkyl amines with allylic carbonates has been achieved. This reaction produces a wide range of chiral homoallylic amines with high enantiopurities. The approach has successfully switched the reactivity between primary alkyl amines and allylic carbonates from intrinsic allylic amination to the α-C−H alkylation, enabling the construction of pharmaceutically significant chiral homoallylic amines from readily available primary alkyl amines in a single step. Chiral amines are widely found in various natural products, bioactive molecules, pharmaceuticals, materials, and catalysts, making them incredibly important [1] , [2] . This has spurred the development of innovative methodologies for synthesizing chiral amines [2] . One of the most effective techniques in organic synthesis is transition-metal-catalyzed asymmetric allylic amination, which could serve as a reliable platform for producing chiral amines [3] , [4] . Primary alkyl amines are a commonly found chemical feedstock. They serve as excellent N-nucleophiles in transition-metal-catalyzed allylic substitution reactions, typically yielding higher-order amines (Fig. 1a ) [3] , [4] . However, if allylic substitution occurs on the α-amino C-H bonds of primary alkyl amines, it would provide a straightforward and intriguing strategy for synthesizing chiral homoallylic amines (Fig. 1a ) [5] . These molecules are not only biologically significant (See Supplementary Fig. 1 in Supplementary Information (SI) for selected examples of bioactive chiral homoallylic amines), but they can also serve as powerful building blocks for constructing nitrogen-containing compounds [6] . However, achieving this transformation is difficult. This is because the acidity of the α-amino C( sp 3 )−H bond is very low (with a p K a estimated to be ~57 by calculation, see SI and Supplementary Data 1 ) [7] , making it challenging to deprotonate it into an active nucleophilic carbanion [8] , [9] . Additionally, the unprotected NH 2 group can seriously interfere with the α-C−H allylic alkylation process (Fig. 1a ). To prevent the interruption of the NH 2 group and facilitate α-C−H deprotonation, protecting group strategies must be employed. The only successful example of such a strategy is reported by Niu et al, where they discover that imines, made from either 9 H -fluoren-9-imine and an alkyl amine [10] or fluoren-9-amine and an alkyl aldehyde [11] , can react with allylic electrophiles in the presence of an iridium catalyst (Fig. 1b ). This reaction forms linear chiral homoallylic amines upon hydrolysis. The reaction proceeds via a pathway involving an Ir-catalyzed allylic substitution on the fluorenyl carbon and subsequent 2-aza-Cope rearrangement, ultimately resulting in formal α-C( sp 3 )−H allylic alkylation of primary amines. The strategy is also effective for activated substrates [12] , [13] , [14] , [15] . Although stoichiometric fluorenone or fluoren-9-amine is used, these elegant studies represent an important early advance in the area. If without protecting group manipulations to the active NH 2 group, direct asymmetric α-C−H allylic alkylation of NH 2 -unprotected primary alkyl amines would be especially synthetically attractive, regarding atom- and step-efficiencies [16] , [17] , [18] , [19] . However, developing this transformation is highly challenging and has not yet been achieved. Fig. 1: α-C−H functionalization of alkyl amines with electrophiles. a N- versus α-C−H allylic alkylation. b Allylic alkylation of alkyl amines through protecting group strategy. c α-C−H Functionalization of activated primary amines through carbonyl catalysis. d This work: asymmetric α-C−H allylic alkylation of primary alkyl amines by synergistic Iridium/ketone catalysis. M metal, L ligand, E + electrophile, cat. catalyst, Me methyl, DBU 1,8-diazabicyclo[5.4.0]undec-7-ene, DFO 1,8-diazafluoren-9-one, THF tetrahydrofuran, ee enantiomeric excess, dr diastereomeric ratio, r.t. room temperature. Full size image Carbonyl catalysis is a process that uses an appropriate aldehyde or ketone to catalyze α-C−H functionalization of primary amines with electrophiles, constructing chiral amines in just one step (Fig. 1c ) [20] , [21] , [22] , [23] , [24] , [25] . Although a series of asymmetric transformations have been achieved by using chiral pyridoxals as carbonyl catalysts [23] , the strategy is mainly limited to activated primary amines such as glycinates [20] , [26] , [27] , benzylamines [28] , and propargylic amines [29] (Fig. 1c ). The reason for this limitation is that primary alkyl amines are highly inert for α-C−H transformation towards electrophiles due to their extremely low acidity (p K a ~ 57). Thus, more powerful carbonyl catalysts are required to activate primary alkyl amines. After considering this challenge, we discover that 1,8-diazafluoren-9-one ( 4 , DFO) [30] can effectively activate primary alkyl amines by forming imines. The acidity of the α-amino C−H bonds is improved by up to 10 44 times, making it acidic enough to be deprotonated under mild conditions (Fig. 1d and Supplementary Fig. 8 ). The strong electron-withdrawing property of the 14π-electron system of the diazafluorene accounts for its extraordinary activating power. Furthermore, in the presence of an iridium catalyst, allylic carbonates can become active electrophiles for allylic alkylation [31] , [32] , [33] , [34] , [35] . Herein, by combining the iridium catalysis and the DFO catalysis [36] , [37] , [38] , [39] , [40] , [41] , [42] , [43] , [44] , [45] , we have successfully achieved direct asymmetric α-C−H allylic alkylation of NH 2 -unprotected primary alkyl amines 1 with allylic carbonates 2 , producing a broad variety of chiral homoallylic amines 3 in good yields with excellent diastereo- and enantioselectivities (up to 95% yield, 98% ee or 99:1 dr) (Fig. 1d ). The reaction undergoes asymmetric allylic substitution on the diazafluorenyl carbon first and then 2-aza-Cope rearrangement, resulting in formal α-C−H allylic alkylation of primary amines without the protection of the strongly nucleophilic NH 2 group [46] . Optimization studies The studies began by searching for efficient carbonyl catalysts that could activate primary alkyl amines (Fig. 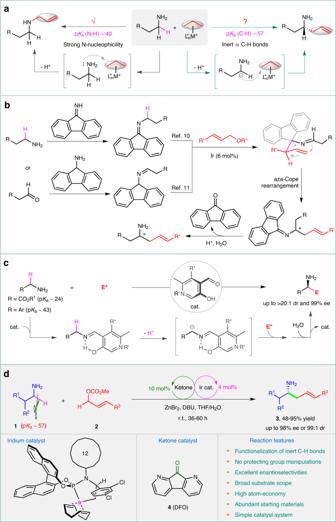Fig. 1: α-C−H functionalization of alkyl amines with electrophiles. aN- versus α-C−H allylic alkylation.bAllylic alkylation of alkyl amines through protecting group strategy.cα-C−H Functionalization of activated primary amines through carbonyl catalysis.dThis work: asymmetric α-C−H allylic alkylation of primary alkyl amines by synergistic Iridium/ketone catalysis. M metal, L ligand, E+electrophile, cat. catalyst, Me methyl, DBU 1,8-diazabicyclo[5.4.0]undec-7-ene, DFO 1,8-diazafluoren-9-one, THF tetrahydrofuran, ee enantiomeric excess, dr diastereomeric ratio, r.t. room temperature. 2 and Supplementary Table 1 ). When the catalyst Ir(COD) 2 BF 4 /( R , R , R a )- L1 was utilized to activate allylic carbonate 2a , several electron-withdrawing aldehydes 5-8 and ketones 4 and 9 were evaluated in the reaction of 2a and primary amine 1a . Only diazafluorenone 4 (DFO) was found to be capable of promoting the desired α-C−H allylic alkylation of 1a , resulting in the formation of chiral homoallylic amine 3a in 87% yield with 92% ee. The Ir(COD) 2 BF 4 /( R , R , R a )- L1 complex controlled the enantioselectivity of the reaction. When phosphoramidite ligand ( R , R a )- L6 was applied, the enantioselectivity was further improved to 97% ee. Without the presence of DFO or iridium catalyst, the α-C−H allylic alkylation did not occur at all (Supplementary Table 1 , entries 1 and 2). It was observed that the addition of a small amount of water to the solvent, tetrahydrofuran, was crucial for enhancing the reaction efficiency (Supplementary Table 1 , entry 32 vs 24). It was believed that water facilitated the hydrolysis of the imine between 3a and 4 , thus accelerating the release of alkylation product 3a and the regeneration of carbonyl catalyst 4 (DFO). In the absence of ZnBr 2 , classic allylic amination occurred predominantly (Supplementary Table 1 , entry 3 vs 4). The additive ZnBr 2 acted as a Lewis acid, promoting the condensation of alkyl amine 1a with diazafluorenone 4 to form an imine that initiated the transformation. Additionally, ZnBr 2 also likely inhibited the undesired allylic amination of 1a by coordinating with the NH 2 group. Fig. 2: Catalyst screening. Reactions were carried out with 1a (0.45 mmol), 2a (0.30 mmol), carbonyl catalyst (0.030 mmol), Ir(COD) 2 BF 4 (0.012 mmol), phosphoramidite ligand (0.0132 mmol), ZnBr 2 (0.45 mmol), and DBU (0.33 mmol) in THF/H 2 O (1.45 mL/0.05 mL) at room temperature for 36 h. During the screening of carbonyl catalysts, phosphoramidite ( R , R , R a )- L1 was used. For the screening of phosphoramide ligands, compound 4 (DFO) was used as the carbonyl catalyst. Isolated yields based on 2a . The ee values were determined by high-performance liquid chromatography (HPLC). a The NMR yields of 3a and 3a’ were determined by 1 H NMR analysis of crude reaction mixtures. Ph phenyl, COD 1,5-cyclooctadiene, NMR nuclear magnetic resonance. Full size image Scope of the reaction Under the optimized conditions, we investigated the substrate scopes of both reaction partners (Fig. 3 ). In the presence of catalytic amounts of Ir(COD) 2 BF 4 /( R , R a )- L6 and diazafluorenone 4 , various cinnamyl (for 3a - n ), naphthyl (for 3o ), heteroaryl (for 3p-q ), and dienyl carbonates (for 3r - t ) smoothly reacted with primary alkyl amine 1a , producing α-substituted chiral amines 3a - t in moderate to high yields (48-95%) with high enantioselectivities (80-97% ee). However, aliphatic allylic carbonates such as ( E )-hex-2-en-1-yl methyl carbonate are ineffective for the α allylic alkylation of primary amines, mainly because the corresponding intermediates generated from the Ir-catalyzed allylic substitution cannot smoothly undergo the 2-aza-Cope rearrangement to form the linear homoallylic amines under the standard conditions. The reaction was also applicable to a broad range of primary alkyl amines. Simple alkyl amines such as ethylamine (for 3v ), n -propylamine (for 3w ), and n -butylamine (for 3u and 3x ), as well as those bearing diverse substituents (for 3ae - ao ), displayed good activity (50–87% yields) and excellent enantioselectivity (91–98% ee) in the reaction. When the smallest primary amine i.e., methylamine was applied to the reaction with ( E )-3-(4-methoxyphenyl)allyl methyl carbonate ( 2b ), a mixture of linear and branched allylic amines, instead of the desired linear homoallylic amines, were obtained as the major products. Secondary amines such as 2-butylamine and cyclohexylamine were inert for the α-C−H allylic alkylation likely due to steric effect and a lower acidity. Primary alkyl amines bearing one or more chiral moieties underwent α-C−H allylic alkylation to afford the corresponding chiral amines 3ap - ba with high diastereoselectivities. Functional groups, such as acetal (for 3ae ), lactam (for 3af ), NHBoc (for 3ak-ao ), OH (for 3ah-aj, 3ap-ar , and 3ba ), and ester ( 3av ), were all well tolerated by the reaction. It is especially impressive that for amino alcohols (for 3ah-aj, 3ap-ar , and 3ba ) containing one or two much more acidic O−H groups, the alkylation still occurred on the highly inert α-C−H bonds. Fig. 3: Substrate scope. The reactions were carried out with 1 (0.45 mmol), 2 (0.30 mmol), 4 (0.030 mmol), Ir(COD) 2 BF 4 (0.012 mmol), ( R , R a )- L6 (0.0132 mmol), ZnBr 2 (0.45 mmol) and DBU (0.33 mmol) in THF/H 2 O (1.45 mL/0.05 mL) at room temperature for 36–60 h unless otherwise stated. Isolated yields were based on carbonates 2 . The ee values were determined by HPLC analysis. The absolute configuration of 3a was determined based on X-ray analysis (Supplementary Fig. 2 ) and those of 3b - ba were tentatively assigned by analogy. a 4 (0.060 mmol) was used. b ( S , S a )- L6 was used. c Reaction in double scale. d Reaction in triple scale. t Bu tert -butyl, Et ethyl, n Pr n -propyl, i Bu iso -butyl, Cy cyclohexyl, Boc tert -butoxycarbonyl. Full size image Synthetic utility The reaction can be scaled up to gram scale, even with a lower catalyst loading (Fig. 4a ). When 2 mol% Ir(COD) 2 BF 4 /( R , R a )- L6 was used, 1.675 g of chiral homoallylic amine 3w was obtained from n -propylamine and allylic carbonate 2b in 82% yield with 93% ee. The products, 3 , which were obtained from the α-C−H allylic alkylation, have demonstrated their synthetic usefulness through various transformations of compound 3w , as shown in Fig. 4a . For instance, hydrogenation of 3w resulted in chiral aliphatic amine 10 in 91% yield. Reaction of 3w with I 2 produced chiral pyrrolidine 11 in 83% yield and 3.7:1 dr, without any loss of enantioselectivity [11] . X-ray analysis confirmed that the major diastereomer was (2 S ,3 R ,5 S )- 11 (Supplementary Fig. 3 ). Treatment of 3w with tert -butyldicarbonate (Boc 2 O), followed by asymmetric dihydroxylation, led to the formation of chiral amino diol 12 with high enantiopurity. Bioactive chiral bicyclic compounds [47] , such as 14 , can also be synthesized in 56% total yield over two steps from compound 3s via intramolecular Diels-Alder reaction. Moreover, the asymmetric α-C−H allylic alkylation can be used for the rapid synthesis of pharmaceuticals. For example, product 3ah underwent condensation with N -carbobenzyloxy-L-alanine, followed by hydrogenation of the C−C double bond and the carbobenzyloxy group, and subsequent condensation with acid 16 , producing anti-Alzheimer’s compound 17 [48] in 88% total yield over three steps. Fig. 4: Synthetic utility and mechanistic studies. a Synthetic applications. b Computational studies. c Proposed mechanism. d Control experiment. e Kinetic isotope effect studies. (DHQD) 2 PHAL bis (dihydroquinidino)phthalazine, Cbz benzyloxycarbonyl, EDCl 1-ethyl−3-(3-dimethylaminopropyl)carbodiimide hydrochloride, HOBt 1-hydroxybenzotriazole, DIPEA diisopropylethylamine. Full size image Mechanistic studies Computational studies have shown that forming imines with diazafluorenone 4 can significantly increase the acidity of the α C−H bonds of alkyl amines, by up to 10 44 times (from p K a 57 of 1c to p K a 12.5 of 18c ) (Fig. 4b ). This increased acidity allows for the deprotonation of the α C−H bonds under mild conditions, producing active 2-azaallyl anions [30] , [49] . Furthermore, the calculated Fukui index reveals that the α‘ carbon of the delocalized carbanion 19c is more nucleophilic than the α carbon [50] , [51] (Fig. 4b ). In addition, Ir-catalyzed allylic substitution reactions typically result in branched products [31] , [32] , [33] , [34] , [35] , [52] , while the current transformation displayed linear regioselectivity. These suggest that the transformation most likely began with Ir-catalyzed allylic substitution, which occurred on the α‘ carbon of the delocalized carbanion 19c , generating a branched intermediate that then underwent aza-Cope rearrangement to form the final linear product 3 , as the pathway of the transformation reported by Niu [10] , [11] . An Iridium/ketone dual catalysis pathway has been proposed (Fig. 4c ). The condensation of alkyl amine 1 with diazafluorenone 4 yields imine 18 , which is deprotonated at the α C−H bond to form 2-azaallyl anion 19 [49] . The delocalized carbanion 19 then undergoes asymmetric addition at the diazafluorenyl carbon to (π-allyl)Ir(III) species 24 , generated from iridium complex 23 and allylic carbonate 2 , resulting in the formation of branched intermediate 21 and the dissociation of the iridium catalyst 23 . Subsequently, compound 21 undergoes 2-aza-Cope rearrangement followed by hydrolysis, leading to α-C−H allylic alkylation product 3 and the regeneration of ketone catalyst 4 . The proposed reaction pathway is in agreement with results from control experiments shown in Fig. 4d , where amine 25 reacted with 3-phenyl propanal to produce imine intermediate 21b , which underwent in situ 2-aza-Cope rearrangement and subsequent hydrolysis to yield amine 3b , the same product obtained from the current α-C−H allylic alkylation of alkyl amine 1a with cinnamyl methyl carbonate (Fig. 4d ). Kinetic isotope effect studies were performed using equimolar amounts of primary alkyl amines 1d and 1d- d (Fig. 4e ). 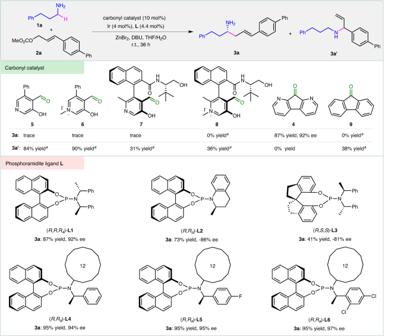Fig. 2: Catalyst screening. Reactions were carried out with1a(0.45 mmol),2a(0.30 mmol), carbonyl catalyst (0.030 mmol), Ir(COD)2BF4(0.012 mmol), phosphoramidite ligand (0.0132 mmol), ZnBr2(0.45 mmol), and DBU (0.33 mmol) in THF/H2O (1.45 mL/0.05 mL) at room temperature for 36 h. During the screening of carbonyl catalysts, phosphoramidite (R,R,Ra)-L1was used. For the screening of phosphoramide ligands, compound4(DFO) was used as the carbonyl catalyst. Isolated yields based on2a. The ee values were determined by high-performance liquid chromatography (HPLC).aThe NMR yields of3aand3a’were determined by1H NMR analysis of crude reaction mixtures. Ph phenyl, COD 1,5-cyclooctadiene, NMR nuclear magnetic resonance. The ratio of products 3ad and deuterated 3ad- d was determined as 6.7:1, indicating that the deprotonation of imine 18 to form active 2-azaallyl carbanion 19 likely is the rate-determining step for the transformation. As shown in the proposed transition state 20 (Fig. 4c ), the chiral environment of the (π-allyl)Ir(III) complex controls the approaching direction of the diazafluorenyl carbanion, determining the absolute configuration of the resulting adduct 21 . The chirality of compound 21 is then transferred to the final product in a stereospecific way via 2-aza-Cope rearrangement, leading to the formation of chiral homoallylic amine 3 in high enantioselectivity. In summary, we have successfully developed a direct asymmetric α-C−H allylic alkylation of NH 2 -unprotected primary alkyl amines through synergistic iridium/ketone catalysis, producing a wide range of chiral homoallylic amines in 48–95% yields with excellent diastereo- and enantioselectivities (up to 98% ee and 99:1 dr) via asymmetric allylic substitution and in situ 2-aza-Cope rearrangement. 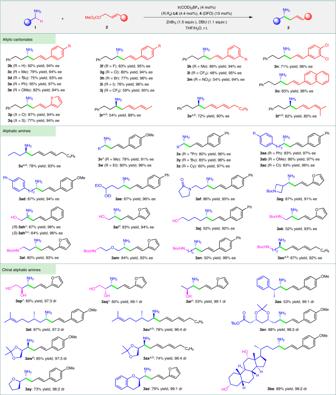Fig. 3: Substrate scope. The reactions were carried out with1(0.45 mmol),2(0.30 mmol),4(0.030 mmol), Ir(COD)2BF4(0.012 mmol), (R,Ra)-L6(0.0132 mmol), ZnBr2(0.45 mmol) and DBU (0.33 mmol) in THF/H2O (1.45 mL/0.05 mL) at room temperature for 36–60 h unless otherwise stated. Isolated yields were based on carbonates2. The ee values were determined by HPLC analysis. The absolute configuration of3awas determined based on X-ray analysis (Supplementary Fig.2) and those of3b-bawere tentatively assigned by analogy.a4(0.060 mmol) was used.b(S,Sa)-L6was used.cReaction in double scale.dReaction in triple scale.tButert-butyl, Et ethyl,nPrn-propyl,iBuiso-butyl, Cy cyclohexyl, Boctert-butoxycarbonyl. 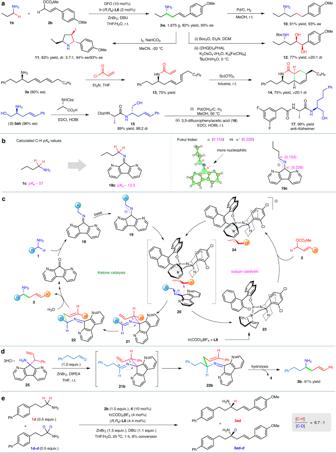Fig. 4: Synthetic utility and mechanistic studies. aSynthetic applications.bComputational studies.cProposed mechanism.dControl experiment.eKinetic isotope effect studies. (DHQD)2PHALbis(dihydroquinidino)phthalazine, Cbz benzyloxycarbonyl, EDCl 1-ethyl−3-(3-dimethylaminopropyl)carbodiimide hydrochloride, HOBt 1-hydroxybenzotriazole, DIPEA diisopropylethylamine. The 1,8-diazafluoren-9-one (DFO) catalyst displays extraordinary power in activating the inert α-C−H bonds of alkyl amines, improving the acidity by up to 10 44 times and leading to the asymmetric α-C−H allylic alkylation. The reaction features excellent stereocontrol, good efficiency and a broad substrate scope, all while avoiding the need for protecting group manipulations and utilizing a simple catalyst system, which provides a straightforward and practical method for synthesizing pharmaceutically significant chiral homoallylic amines, from readily available alkyl primary amines. General procedure for catalytic asymmetric α-C( sp 3 )−H allylic alkylation In a glove box, to a dry 5-mL vial equipped with a magnetic stirrer bar were added Ir(COD) 2 BF 4 (5.9 mg, 0.012 mmol), ( R,R a )- L6 (8.8 mg, 0.0132 mmol), THF (0.20 mL) and primary amine 1 (0.15 mmol) (Note: Introducing a part of the primary amine 1 during the catalyst preparation is helpful for accelerating the formation of the active Ir catalyst) [53] . The vial was sealed and taken out of the glove box. The mixture was stirred at 50 o C for 30 min and then cooled down to room temperature, which was used as the solution of the Ir catalyst. In the glove box, to a 10 mL Schlenk tube equipped with a magnetic stirrer bar were added 1,8-diazafluoran-9-one ( 4 , DFO) (5.5 mg, 0.030 mmol), THF (0.20 mL), primary amine 1 (0.30 mmol) and a solution of ZnBr 2 (0.101 g, 0.45 mmol) in THF (0.30 mL). The Schlenk tube was sealed and taken out of the glove box. After being stirred at room temperature for 30 min, to the mixture were added allylic carbonate 2 (0.30 mmol, dissolved in 0.40 mL dry THF), 1,8-diazabicyclo[5.4.0]undec-7-ene (DBU) (0.050 g, 0.33 mmol), the pre-prepared solution of the Ir catalyst, THF (0.35 mL) and water (0.050 mL). The reaction mixture was stirred at room temperature for 36 h. A hydroxylamine (NH 2 OH) aqueous solution (0.050 mL, 50 wt% in water) was added to quench the reaction. After stirring at room temperature for 1 h, ammonium hydroxide solution (5.0 mL, 25–28 wt% in water) was added and the resulting mixture was extracted with DCM (20 mL × 3). The combined organic layers were dried over Na 2 SO 4 , filtered, concentrated under reduced pressure and purified via column chromatography on silica gel (ethyl acetate: dichloromethane: triethylamine = 100:10:1, the silica gel column was eluted with 1% v/v solution of Et 3 N in petroleum ether before sample loading) to afford compound 3 . For some specific substrates, the reaction conditions were slightly changed, the detailed information of which can be found in the SI.